Evidence that breast cancer risk at the 2q35 locus is mediated throughIGFBP5regulation GWAS have identified a breast cancer susceptibility locus on 2q35. Here we report the fine mapping of this locus using data from 101,943 subjects from 50 case-control studies. We genotype 276 SNPs using the ‘iCOGS’ genotyping array and impute genotypes for a further 1,284 using 1000 Genomes Project data. All but two, strongly correlated SNPs (rs4442975 G/T and rs6721996 G/A) are excluded as candidate causal variants at odds against >100:1. The best functional candidate, rs4442975, is associated with oestrogen receptor positive (ER+) disease with an odds ratio (OR) in Europeans of 0.85 (95% confidence interval=0.84−0.87; P=1.7 × 10 −43 ) per t -allele. This SNP flanks a transcriptional enhancer that physically interacts with the promoter of IGFBP5 (encoding insulin-like growth factor-binding protein 5) and displays allele-specific gene expression, FOXA1 binding and chromatin looping. Evidence suggests that the g -allele confers increased breast cancer susceptibility through relative downregulation of IGFBP5, a gene with known roles in breast cell biology. The 2q35 breast cancer locus was originally identified in an Icelandic genome-wide association study (GWAS) [1] , and subsequently confirmed in larger European studies. The largest replication study, comprising 25 studies from the Breast Cancer Association Consortium, yielded odds ratio (OR) of 0.89 (95% CI −0.87 to 0.92) per g -allele for rs13387042 with evidence for association with both oestrogen receptor-positive (ER+) and ER-negative (ER−) disease [2] . rs13387042 lies in a 210-kb linkage disequilibrium (LD) block within a gene ‘desert’, bounded centromerically by the transition nuclear protein 1 gene ( TNP1 —181 kb proximal) and telomerically by the disrupted in renal carcinoma 3 gene ( DIRC3 —243 kb distal). Additional but more distant centromeric genes are two members of the insulin growth factor-binding protein family, IGFBP5 (345 kb proximal) and IGFBP2 (376 kb proximal). In the current study, we describe the fine-scale mapping of the 2q35 breast cancer susceptibility locus using 1,560 genotyped and imputed single nucleotide polymorphisms (SNPs) in 101,943 subjects from 50 case-control studies. The strongest candidate for causality, SNP rs4442975, flanks a transcriptional enhancer that physically interacts with the promoter of IGFBP5 . Furthermore, we demonstrate that rs4442975 is associated with allele-specific FOXA1 binding, chromatin looping and IGFBP5 expression. Our data suggest that the g -allele of rs4442975 confers increased breast cancer susceptibility through reduced IGFBP5 expression. Fine-scale mapping identifies two candidate causal variants Association analyses were performed on 1,560 2q35 SNPs (276 genotyped and 1,284 imputed at r 2 >0.3). Three hundred and fifty-two SNPs are associated with overall breast cancer, 327 with ER+ and none with ER− breast cancer ( P values <10 −4 ; Supplementary Data 1 ) in European-ancestry women. The genotyped SNP rs4442975 displays the strongest association (per- t -allele OR=0.87; 95% CI −0.86 to 0.89; P= 3.9 × 10 −46 ; Fig. 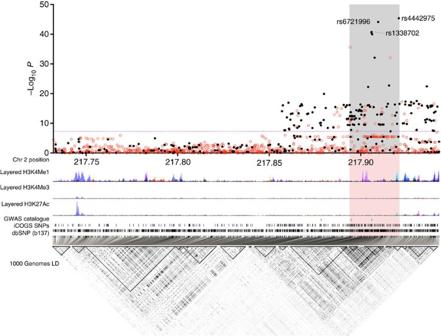Figure 1: Genetic mapping and epigenetic landscape at the 2q35 locus. Manhattan plot of the 2q35 breast cancer susceptibility locus. Genotyped (black dots) and imputed (red dots) SNPs are plotted based on their chromosomal position on thexaxis and their overallPvalues (log10values, likelihood ratio test) from the European BCAC studies (46,451 cases and 42,599 controls) on theyaxis. The shaded region represents an area bounded by SNPs correlated with rs4442975 atr2=0.8. Data from the UCSC Genome Browser, including epigenetic marks for methylation of histone H3 at lysine 4 (H3K4me1, H3K4me3) and acetylation of H3 at lysine 27 (H3K27ac) in seven cell types from ENCODE28. The positions of all analysed iCOGS SNPs are marked. LD, using data from the BCAC population, is depicted beneath—white representsr2=0 and blackr2=1. 1 ; Table 1 ; Supplementary Fig. 1 ) and this is stronger for ER+ disease (OR=0.85; 95% CI −0.84 to 0.87; P= 1.69 × 10 −43 ) than for ER− disease (OR=0.95; 95% CI −0.91 to 0.98; P= 0.0043; P heterogeneity=2.8 × 10 −6 ; Table 1 ). Figure 1: Genetic mapping and epigenetic landscape at the 2q35 locus. Manhattan plot of the 2q35 breast cancer susceptibility locus. Genotyped (black dots) and imputed (red dots) SNPs are plotted based on their chromosomal position on the x axis and their overall P values (log 10 values, likelihood ratio test) from the European BCAC studies (46,451 cases and 42,599 controls) on the y axis. The shaded region represents an area bounded by SNPs correlated with rs4442975 at r 2 =0.8. Data from the UCSC Genome Browser, including epigenetic marks for methylation of histone H3 at lysine 4 (H3K4me1, H3K4me3) and acetylation of H3 at lysine 27 (H3K27ac) in seven cell types from ENCODE [28] . The positions of all analysed iCOGS SNPs are marked. LD, using data from the BCAC population, is depicted beneath—white represents r 2 =0 and black r 2 =1. Full size image Table 1 Association of the two most strongly associated SNPs (rs4442975 and rs6721996) and the original GWAS SNP (rs13387042) with breast cancer. Full size table We next conducted multivariable logistic regression for both overall and ER+ breast cancer, examining each SNP with univariate P <10 −4 ( N =330) in an analysis adjusted for the most significant SNP rs4442975. No further variants are strongly associated with overall or ER+ disease. The second most strongly associated SNP for overall breast cancer after adjusting for rs4442975 is rs10191184 (OR=0.96; 95% CI=0.93 to 0.99; P= 0.0048), consistent with the hypothesis of a single causative variant. We compared the log likelihoods from the ER+ univariate regression models for each SNP with the log likelihood for rs4442975. All SNPs except one (rs6721996), which was almost perfectly correlated with rs4442975 ( r 2 =0.98), have log likelihoods >100 times lower than rs4442975 and hence can reasonably be excluded as being causative. The excluded variants include the original GWAS hit, rs13387042, which is strongly correlated with rs4442975 ( r 2 =0.93) but has odds of 3300:1 against being causative ( Table 1 ). Haplotype analyses of the five most strongly associated SNPs identified two common and one rarer haplotype (frequency 1.4%: Supplementary Table 1 ). The rare haplotype (1) carries the cancer-protective alleles at rs4442975 ( t- allele) and rs6721996 ( a -allele), but not rs13387042, and has a similar risk to haplotype 2, carrying the protective alleles at all five SNPs, which is consistent with the hypothesis of rs4442975 and/or rs6721996 being the causal variant. In Asian studies, the protective alleles for both candidate causal variants (rs4442975 and rs6721996) are rarer (minor allele frequencies (MAFs)=0.13 and 0.12, respectively) than in Europeans (MAF=0.49) but their associated relative risk estimates with overall breast cancer are consistent: per t -allele OR (rs4442975)=0.94; 95% CI −0.87 to 1.02; P= 0.12 and per a -allele OR (rs6721996)=0.95; 95% CI −0.88 to 1.03; P= 0.20 ( Table 1 ). rs4442975 resides near a putative regulatory element We used available ENCODE chromatin immunoprecipitation-sequencing (ChIP-seq) data to map the candidate causal SNPs relative to transcriptional regulatory elements. SNP rs4442975 lies near a putative regulatory element (PRE) as defined by H3K4Me1 histone modifications in seven cell types from ENCODE, and H3K4Me2 in MCF7 cells ( Figs 1 and 2a ). This PRE also contains DNaseI-hypersensitive sites in both MCF7 and HMEC cell lines (indicative of regions of open chromatin) and binds several transcription factors (TFs) associated with oestrogen signalling [3] ( Fig. 2a ). By contrast, the region surrounding SNP rs6721996 does not contain specific histone modifications or relevant TF binding in the cell lines analysed ( Fig. 2a ). 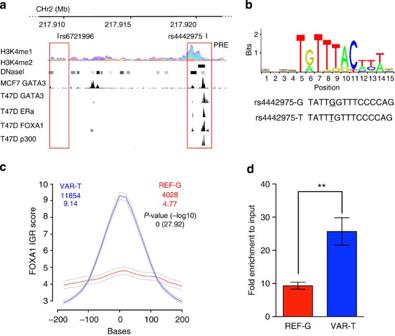Figure 2: Allele-specific binding of FOXA1 at the rs4442975 site. (a) Epigenetic and transcriptional landscape of the 2q35 risk interval. Coloured histogram denotes histone modification ChIP-seq data from ENCODE. Data from the UCSC Genome Browser, including epigenetic marks for H3K4me1 in seven cell types from ENCODE28, H3K4me2 from MCF7 cells4, DNaseI hypersensitivity clusters in 125 cell types from ENCODE28, and TF ChIP-seq data from MCF7 and T47D ER+ breast cancer cells, which are homozygous for theg-allele of rs4442975 and rs6721996 (ENCODE). The PRE contains SNP rs4442975. (b) Position weight matrix of FOXA1 from JASPAR, with homology to the risk (g) and cancer-protective (t) alleles of rs4442975 coloured below. (c) IGR histogram for SNP rs4442975 predicting the binding intensity of FOXA1 using a seven-nucleotide affinity model5. The top row of coloured numbers shows the number of instances for each K-mer found genome wide within H3K4me2 elements in MCF7 cells. The bottom row shows the averaged binding intensities at the K-mers (50 bp window). Control profiles, shown in grey, are generated by scrambling the probed sequence. (d) Allele-specific FOXA1 ChIP-qPCR results assessed at the rs4442975 SNP in heterozygous BT474 breast cancer cells. Error bars denote s.d.Pvalues were determined with a two-tailedt-test. **P<0.01. Figure 2: Allele-specific binding of FOXA1 at the rs4442975 site. ( a ) Epigenetic and transcriptional landscape of the 2q35 risk interval. Coloured histogram denotes histone modification ChIP-seq data from ENCODE. Data from the UCSC Genome Browser, including epigenetic marks for H3K4me1 in seven cell types from ENCODE [28] , H3K4me2 from MCF7 cells [4] , DNaseI hypersensitivity clusters in 125 cell types from ENCODE [28] , and TF ChIP-seq data from MCF7 and T47D ER+ breast cancer cells, which are homozygous for the g -allele of rs4442975 and rs6721996 (ENCODE). The PRE contains SNP rs4442975. ( b ) Position weight matrix of FOXA1 from JASPAR, with homology to the risk ( g ) and cancer-protective ( t ) alleles of rs4442975 coloured below. ( c ) IGR histogram for SNP rs4442975 predicting the binding intensity of FOXA1 using a seven-nucleotide affinity model [5] . The top row of coloured numbers shows the number of instances for each K-mer found genome wide within H3K4me2 elements in MCF7 cells. The bottom row shows the averaged binding intensities at the K-mers (50 bp window). Control profiles, shown in grey, are generated by scrambling the probed sequence. ( d ) Allele-specific FOXA1 ChIP-qPCR results assessed at the rs4442975 SNP in heterozygous BT474 breast cancer cells. Error bars denote s.d. P values were determined with a two-tailed t -test. ** P <0.01. Full size image rs4442975 alters FOXA1 DNA binding Breast cancer susceptibility loci have been shown to be enriched for FOXA1-binding sites at active regulatory elements in breast cancer cells; and the 2q35 locus contains variants predicted to modulate the affinity of FOXA1 (ref. 4 ). FOXA1 is a pioneer factor and master regulator of ER activity due to its ability to open local chromatin and recruit ER to target gene promoters [5] , [6] . SNP rs4442975 is predicted, in silico , to lie in a FOXA1-binding site with the t -allele promoting increased FOXA1 binding compared with the g -allele ( Fig. 2b,c ; Supplementary Fig. 2 ). To assess occupancy of FOXA1 in vivo , we conducted ChIP followed by allele-specific quantitative PCR (qPCR) in the heterozygous BT474 breast cancer cell line. We found that FOXA1 is indeed preferentially recruited to the t (cancer-protective) allele of candidate causal SNP rs4442975 ( Fig. 2d ; Supplementary Fig. 3 ). Of note, ChIP-seq data from ENCODE identified a second, albeit weaker, FOXA1-binding motif upstream of rs4442975 that may also influence FOXA1 recruitment ( Fig. 2a ). However, ChIP-qPCR did not detect FOXA1 binding in vivo to this additional site, and due to the limited availability of FOXA1-positive breast cancer cell lines with the relevant genotypes, we are unable to unequivocally discern its affinity for FOXA1. Consequently, while our results support a role for rs4442975 in modulating FOXA1-binding affinity on the site of overlap, we cannot exclude additional cis -effects typical of multi-enhancer variants [7] where a rare variant, yet to be identified, would be in LD with rs4442975 and influence the recruitment of FOXA1 or other factors found in the same LD block. rs4442975 interacts with the IGFBP5 promoter To determine the target gene(s), we used chromatin conformation capture (3C), which revealed that the PRE containing rs4442975 frequently interacts with the IGFBP5 promoter (located 345 kb proximal) in both ER+ breast cancer cell lines (MCF7 and BT474) and in normal breast epithelial cells (MCF10A and Bre-80; Fig. 3a ). No significant interactions were detected between this PRE and other flanking genes including IGFBP2 , XRCC5 , TNP1 and DIRC3 ( Fig. 3a ; Supplementary Figs 4–7 ). The region surrounding SNP rs6721996 did not interact with any flanking genes including the IGFBP5 promoter ( Supplementary Figs 4–7 ). To assess any potential impact of SNP rs4442975 on this chromatin interaction, allele-specific 3C was performed in heterozygous BT474 cell lines. Sequence profiles indicate that the rs4442975 t -allele is more strongly associated with looping of this PRE to the IGFBP5 promoter than the g -allele ( Fig. 3b ; Supplementary Fig. 8 ), suggesting that the cancer-protective t -allele may increase IGFBP5 expression through preferential contact between this element and the IGFBP5 promoter. 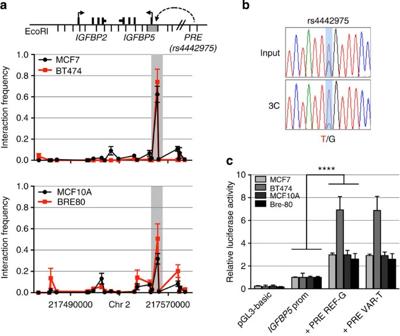Figure 3: Chromatin interactions at the 2q35 risk region withIGFBP5in breast cell lines. (a) 3C interaction profiles between the PRE (containing rs4442975) and theIGFBP5promoter region (grey box). 3C libraries were generated with EcoRI, with the anchor point set at the PRE. A physical map of the region interrogated by 3C is shown above, with the grey bar representing the position of theIGFBP5promoter (not to scale). Graphs represent three biological replicates assayed in duplicate. Error bars denote s.d. (b) 3C followed by sequencing for the rs4442975-containing region in heterozygous BT474 breast cancer cells shows allele-specific chromatin looping. Chromatograms represent one of the three independent 3C libraries generated and sequenced. (c) Luciferase reporter assays in breast cell lines demonstrating enhancer activity of the PRE at the 2q35 risk locus. The PRE was cloned upstream of anIGFBP5promoter-driven luciferase reporter with and without SNP rs4442975. Cells were transiently transfected with each of these constructs and assayed for luciferase activity after 24 h. Graphs represent two independent experiments assayed in triplicate. Error bars denote s.d.Pvalues were determined with a two-tailedt-test. ****P<0.0001. Figure 3: Chromatin interactions at the 2q35 risk region with IGFBP5 in breast cell lines. ( a ) 3C interaction profiles between the PRE (containing rs4442975) and the IGFBP5 promoter region (grey box). 3C libraries were generated with EcoRI, with the anchor point set at the PRE. A physical map of the region interrogated by 3C is shown above, with the grey bar representing the position of the IGFBP5 promoter (not to scale). Graphs represent three biological replicates assayed in duplicate. Error bars denote s.d. ( b ) 3C followed by sequencing for the rs4442975-containing region in heterozygous BT474 breast cancer cells shows allele-specific chromatin looping. Chromatograms represent one of the three independent 3C libraries generated and sequenced. ( c ) Luciferase reporter assays in breast cell lines demonstrating enhancer activity of the PRE at the 2q35 risk locus. The PRE was cloned upstream of an IGFBP5 promoter-driven luciferase reporter with and without SNP rs4442975. Cells were transiently transfected with each of these constructs and assayed for luciferase activity after 24 h. Graphs represent two independent experiments assayed in triplicate. Error bars denote s.d. P values were determined with a two-tailed t -test. **** P <0.0001. Full size image rs4442975 influences IGFBP5 expression The regulatory capability of the PRE, combined with the effect of SNP rs4442975, was further examined in luciferase reporter assays, using constructs containing the IGFBP5 promoter. The wild-type PRE acts as a transcriptional enhancer, leading to a 2–3 fold increase in IGFBP5 promoter activity ( Fig. 3c ; PRE REF-G), but inclusion of the rs4442975 t -allele has no significant effect on the PRE enhancer activity ( Fig. 3c ; PRE REF-T). While this appears to rule out an effect of this SNP on transactivation, it is possible that rs4442975 is influencing gene expression through other regulatory mechanisms. To assess the impact of the rs4442975 alleles on IGFBP5 expression, we measured endogenous levels of IGFBP5 mRNA in ER-positive breast cancer cell lines either homozygous (G/G) or heterozygous (G/T) for SNP rs4442975. While limited in number, the results showed that IGFBP5 mRNA was significantly increased in heterozygous cell lines ( Fig. 4a ). Furthermore, given the importance of FOXA1 in oestrogen–ER activity, we also measured endogenous levels of IGFBP5 mRNA in MCF7 (G/G) and BT474 (G/T) cells following oestrogen induction and found that IGFBP5 mRNA was significantly increased but only in the heterozygous BT474 cells ( Fig. 4b ; Supplementary Fig. 9 ). To evaluate allele-specific IGFBP5 expression, we identified a heterozygous variant (pos271557291) in the first intron of IGFBP5 in BT474 cells. Sequencing of the 3C product showed that the t -allele of rs4442975 is physically linked to the variant c -allele of pos271557291 ( Supplementary Fig. 10 ). Allele-specific expression assays revealed that the c -allele of variant pos271557291 is preferentially expressed, supporting our conclusion that the protective t -allele of rs4442975 is associated with an increase in IGFBP5 expression ( Fig. 4c ; Supplementary Fig. 11 ). 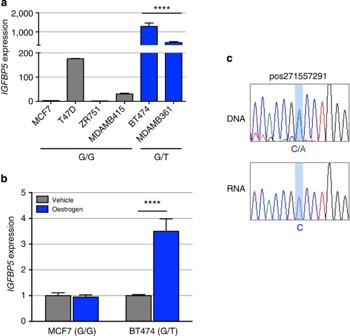Figure 4:IGFBP5expression in breast cancer cell lines and normal breast tissue. (a) EndogenousIGFBP5expression measured by qPCR in untreated ER+ human breast cancer cell lines and (b) oestrogen-stimulated breast cancer cell lines. Graphs represent three independent experiments. Error bars denote s.e.m.Pvalues were determined by a two-tailedt-test. ****P<0.0001. (c) Allele-specificIGFBP5expression measured by allelic amplification of intronic marker variant pos271557291. Chromatograms represent one of the three independent experiments performed and sequenced. Figure 4: IGFBP5 expression in breast cancer cell lines and normal breast tissue. ( a ) Endogenous IGFBP5 expression measured by qPCR in untreated ER+ human breast cancer cell lines and ( b ) oestrogen-stimulated breast cancer cell lines. Graphs represent three independent experiments. Error bars denote s.e.m. P values were determined by a two-tailed t -test. **** P <0.0001. ( c ) Allele-specific IGFBP5 expression measured by allelic amplification of intronic marker variant pos271557291. Chromatograms represent one of the three independent experiments performed and sequenced. Full size image Gene expression analyses in breast tissue Finally, we examined the associations of rs4442975 with expression levels of genes within 1 Mb of the SNPs, in 123 normal breast tissue samples and 254 breast tumour samples in the Norwegian Breast Cancer Study (NBCS), and additionally in 135 normal breast tissue samples from the Molecular Taxonomy of Breast Cancer International Consortium (METABRIC) study. In normal breast tissue from NBCS, SNP rs4442975 is associated with expression levels of the IGFBP5 probe, A_23_P154115 ( P= 0.045), and similarly in METABRIC with the IGFBP5 probe, ilmn_1750324 ( P =0.026; Supplementary Table 2 ), but there are no associations with other IGFBP5 probes used in these studies. In both studies, the protective t -allele of rs4442975 was associated with slightly increased IGFBP5 levels ( Supplementary Fig. 12 ). However, for each tested IGFBP5 probe there are other more strongly expression-associated SNPs (eSNPs) at this locus, none of which are significantly correlated with the breast cancer risk candidate SNP, rs4442975 ( r 2 <0.001; Supplementary Table 2 ). No significant associations were observed between rs4442975 and expression of any other genes in NBCS normal breast tissues or breast tumours, nor in METABRIC normal breast samples ( Supplementary Table 3 ). In this study, we have conducted a comprehensive analysis of all known common variants within a 210-kb interval of the original 2q35 locus. We identified one independent set of correlated, highly trait-associated variants (iCHAV) [8] for ER-positive breast cancer. Our data are consistent with a single disease-associated variant, with no evidence for further SNPs being associated with breast cancer risk after adjustment for the candidate causal SNP, rs4442975. However, we recently identified another iCHAV for breast cancer >300 Kb telomeric to rs4442975 (ref. 9 ). These two iCHAVs are separated by several recombination hotspots, and their tagging SNPs are uncorrelated ( r 2 =0.002). This observation fits the general pattern that multiple independent cancer susceptibility variants fall within GWAS-identified loci [7] , [10] , and raises the possibility that both associations are mediated through the same target gene. Our allele-specific 3C and expression analyses provided evidence that rs4442975 contributes to changes in IGFBP5 expression. Although not robustly supported by our expression quantitative trait locus (eQTL) studies, two independent data sets showed that the protective t -allele of rs4442975 was associated with slightly increased IGFBP5 levels, which is consistent with our functional results. However, we also identified other eSNPs in the region that are more strongly associated with IGFBP5 expression in normal breast tissue, but do not drive breast cancer risk. This situation is not dissimilar to other loci we have studied, where we have not found that the causal risk SNPs are strong eQTLs for the gene they regulate [11] , [12] , [13] . This disparity may at least partly be explained by the fact that eSNPs are acting in multiple tissues, but risk-associated SNPs may only act in one specific cell type. Given that normal breast tissue is so heterogeneous, any eQTL effect that is specific to one cell type (such as stem cells) is going to be significantly diluted. In addition, eQTLs are very context dependent, so might only be expressed in breast tissue under particular stimuli or stages of development. It is also possible that the relevant cells for the analysis are luminal progenitor cells in adolescence, when the human breast seems susceptible to environmental and hormonal influences, but we have no access to data from them. The best understood activity of the IGFBPs is sequestration of extracellular IGFs to control their growth-promoting actions. IGFBP5, which is expressed in both normal and cancer tissues, is a key member of this IGF axis—regulating cellular growth, differentiation and apoptosis [14] , [15] , but IGF-independent actions of IGFBP5 have also been demonstrated in various cell types [16] , [17] . The roles of IGFBP5 in human breast cancer are complex and there are many contradictory findings: some lines of evidence suggest that IGFBP5 acts as an inhibitor of tumour growth. For example, Butt et al. [18] reported that increased expression of IGFBP5 inhibits human breast cancer cell growth. Consistent with a pro-apoptotic effect, transgenic mice, expressing IGFBP5 in mammary gland, have impaired mammary development and increased apoptotic cell death [19] . Other evidence indicates, conversely, that IGFBP5 has anti-apoptotic and tumour-promoting actions; Perks et al. [20] reported that exogenous IGFBP5 inhibits apoptosis of breast cancer cells in vitro . Very low IGFBP5 expression has been detected in benign breast epithelium with high expression levels in adjacent breast tumour tissue [21] , [22] . We propose that the g -allele of SNP rs4442975 (associated with increased risk) reduces FOXA1 binding and hence results in reduced chromatin accessibility, cofactor recruitment and long-range chromatin interactions. Taken together, all these lines of evidence point to increased breast cancer risk, associated with the rs4442975 g -allele, being mediated through reduced IGFBP5 expression. The IGF axis is already an important therapeutic target in other human cancers [23] , and our findings suggest further studies on IGFBP5 and breast cancer prevention may be merited. Study populations and genotyping Epidemiological data were obtained from 50 breast cancer case-control studies participating in the Breast Cancer Association Consortium; these comprised 41 studies from populations of European ancestry and 9 studies from populations of East Asian ancestry [9] . Genotyping was conducted using the iCOGS array, a custom array comprising ~200,000 SNPs. Details of the participating studies, genotyping calling and quality control are given elsewhere [9] . After quality control exclusions, we analysed data from 46,451 cases and 42,599 controls of European ancestry and 6,269 cases and 6,624 controls of Asian ancestry. ER status of the primary tumour was available for 34,539 European and 4,972 Asian cases; of these 7465 (22%) European and 1610 (32%) Asian cases were ER negative [9] . SNP selection and genetic mapping We first defined a mapping interval of 210,596 bp (positions 217, 732, 119–217, 942, 715; NCBI build 37 assembly) based on the LD block that included rs13387042 in Hapmap (CEU). We catalogued 1,578 variants in the region using the 1000 Genomes Project (March 2010 Pilot version 60 CEU project data), of which 751 variants had a MAF >2%. Of these, we selected all SNPs correlated with the rs13387042 at r 2 >0.1 ( N =150), plus a set of SNPs designed to tag all remaining SNPs with r 2 >0.9 ( N =137). All but 11 SNPs passed a designability score (DS) provided by Illumina (DS>0.9) and were included on the iCOGS array. The 276 SNPs included on the array all passed quality control and were included in this analysis. The genotype data were then used to impute genotypes at all additional known SNPs in the interval using IMPUTE version 2.0 and the 1000 Genome Project data (March 2012 version) as a reference panel. One thousand two hundred and eighty-four variants were successfully imputed, with imputation r 2 >0.3 in Europeans. Statistical analysis Per-allele ORs and s.e. were estimated for each SNP using logistic regression, separately for subjects of European and Asian ancestry, and separately for overall, ER-positive and ER-negative breast cancer. The association between each SNP and breast cancer risk was tested using a one-degree-of-freedom trend test adjusted for study and seven principal components. The statistical significance of each SNP was derived using a Wald test. To evaluate evidence for multiple association signals, we performed conditional analyses, in which the association for each SNP was re-evaluated after including other associated SNPs in the model. SNPs with a P value <10 −4 and MAF >2% in the single SNP analysis were included in this analysis [9] . Differences in the OR between ER-positive and ER-negative disease were assessed using a case-only analysis, with ER status as the dependent variable. Haplotype-specific ORs and confidence limits were estimated using haplo.stats [24] . Cell lines and treatments Breast cancer cell lines MCF7 (ER+; ATCC #HTB22), T47D (ER+; ATCC #HTB-133), ZR751 (ER+; ATCC #CRL-1500), MDAMB415 (ER+; ATCC #HTB-128) and BT474 (ER+; ATCC #HTB20) were grown in RPMI medium with 10% fetal calf serum and antibiotics. MDAMB361 (ER+; kindly provided by Sunil Lakhani, UQCCR, Brisbane) were grown in DMEM with 20% fetal calf serum and antibiotics. Normal breast epithelial cell lines MCF10A (ATCC #CRL 10317) and Bre-80 (kindly provided by Roger Reddel, CMRI, Sydney) were grown in DMEM/F12 medium with 5% horse serum, 10 μg ml −1 insulin, 0.5 μg ml −1 hydrocortisone, 20 ng ml −1 epidermal growth factor and 100 ng ml −1 cholera toxin and antibiotics. For oestrogen induction, 24 h after plating MCF7 or BT474 cells into 24-well plates, medium was replaced with that containing 10 nM fulvestrant. Cells were incubated for 48 h and then fresh medium containing either 10 nM oestrogen or DMSO (dimethylsulphoxide; as vehicle control) was added [25] . All cell lines were maintained under standard conditions, routinely tested for Mycoplasma and identity profiled with short tandem repeat markers. Chromatin conformation capture (3C) Breast cancer cell lines were grown to 80% confluence, then crosslinked with 1% formaldehyde at 37 °C for 10 min, quenched with ice-cold 125 mM glycine and collected by cell scraping. Cells were then washed twice in ice-cold phosphate-buffered saline (PBS), lysed for 30 min on ice in 10 ml lysis buffer (10 mM Tris-HCl, pH 7.5, 10 mM NaCl, 0.2% Igepal, 1 × protease inhibitor cocktail) and homogenized with 15 strokes in a Dounce homogenizer. Nuclei were then pelleted for 10 min (800 g at 4 °C), washed in PBS and resuspended in 1 ml 1.2 × EcoRI restriction buffer and 0.3% SDS for 1 h at 37 °C with shaking. Triton X-100 (2%) was added to sequester SDS, and then each tube was digested with 1,500 U EcoRI for 24 h at 37 °C with shaking. One aliquot of digested cells was set aside to assess restriction enzyme efficiency by real-time PCR (qPCR), the rest was ligated with 4,000 U of T4 DNA ligase for 4 h at 16 °C. Crosslinks were reversed by proteinase K digestion overnight, and then the 3C DNA template was purified by phenol–chloroform extraction followed by four rounds of ethanol precipitation. The final DNA pellet was dissolved in 10 mM Tris (pH 7.5) overnight at 4 °C, purified through Amicon Ultra 0.5 ml columns (EMD Millipore) and quantitated by qPCR. 3C interactions were quantitated by qPCR using primers designed within EcoRI restriction fragments ( Supplementary Table 4 ). All qPCRs were performed on a RotorGene 6000 using MyTaq HS DNA polymerase with the addition of 5 mM of Syto9, annealing temperature of 66 °C and extension of 30 s. 3C analyses were performed in three independent experiments with each experiment quantified in duplicate. BAC clones (RP11-96E20, RP11-944D16, RP11-14F16, RP11-639B13, RP11-43F9, RP11-22K2) covering the 2q35 region were used to create artificial libraries of ligation products to normalize for PCR efficiency. Data were normalized to the signal from the BAC clone library and, between cell lines, by reference to a region within GAPDH . All qPCR products were electrophoresed on 2% agarose gels, gel purified and sequenced to verify the 3C product. Plasmid construction and luciferase assays The IGFBP5 promoter-driven luciferase reporter construct was generated by inserting a 1,071-bp fragment containing the IGFBP5 promoter into the KpnI and XhoI sites of pGL3-basic. To assist cloning, AgeI and SbfI sites were inserted into the BamHI and SalI sites downstream of luciferase. A 1,296-bp fragment containing the PRE was inserted into the AgeI and SbfI sites downstream of luciferase. SNP rs4442975 was incorporated into the PRE using overlap extension PCR. All constructs were sequenced to confirm variant incorporation (AGRF, Australia). Primers used to generate all constructs are listed in Supplementary Table 4 . MCF7, BT474, MCF10A and Bre-80 breast cells were transfected with equimolar amounts of luciferase reporter plasmids and 50 ng of pRLTK using Lipofectamine 2000. The total amount of transfected DNA was kept constant per experiment by adding carrier plasmid (pUC19). Luciferase activity was measured 24 h post transfection using the Dual-Glo Luciferase Assay System on a Beckman-Coulter DTX-880 plate reader. To correct for any differences in transfection efficiency or cell lysate preparation, Firefly luciferase activity was normalized to Renilla luciferase. The activity of each test construct was calculated relative to IGFBP5 promoter construct, the activity of which was arbitrarily defined as 1. Intragenomic replicates Intragenomic replicates (IGR) predicts the modulation in affinity produced by a SNP at a TF-binding site [4] . The affinity of a TF for a particular DNA sequence of length K (K-mer) is obtained by averaging binding data across a ChIP-seq data set for that TF. IGR accounts for displacement effects by computing affinity models over a sliding window of K-mers around the SNP of interest. Through this process, the collection of affinity models for increasing values of K is placed in a lattice structure that connects K-mers, which are 1 bp apart. Two lattices are constructed, one for each of the variants alleles. The maxima among the affinity models in the lattices is used to calculate the IGR score. T -tests are used to assess the statistical significance of the affinity modulation between the two K-mers with the maximum affinities. Allele-specific ChIP-qPCR Breast cancer cell lines were grown to 95% confluence, crosslinked with 1% formaldehyde at 37 °C for 10 min, cells were rinsed with ice-cold PBS plus 5% bovine serum albumin and then with PBS and collected with PBS plus 1 × protease inhibitor cocktail (Roche Molecular Biochemicals, Indianapolis, IN). Collected cells were centrifuged for 2 min at 3,000 r.p.m. Cell pellet was then resuspended in 0.35 ml of lysis buffer (1% SDS, 10 mM EDTA, 50 mM Tris-HCl, pH 8.1, 1 × protease inhibitor cocktail) and sonicated 20 times in 30 s on 30 s off cycles at the maximum setting (Diagenode Biorupter 300) followed by centrifugation at maximum speed for 15 min. Supernatants were collected and diluted in dilution buffer (1% Triton X-100, 2 mM EDTA, 150 mM NaCl, 20 mM Tris-HCl, pH 8.1). Four micrograms of FOXA1 antibody (Acris, AP16139PU-N) was prebound for 6 h to protein A and protein G Dynal magnetic beads (Dynal Biotech, Norway) and washed three times with ice-cold PBS plus 5% bovine serum albumin and then added to the diluted chromatin for overnight immunoprecipitation. The magnetic bead–chromatin complexes were collected and washed six times in RIPA buffer (50 mM HEPES (pH 7.6), 1 mM EDTA, 0.7% Na deoxycholate, 1% NP-40, 0.5 M LiCl), then washed twice with Tris-EDTA buffer. To reverse the formaldehyde crosslinking, decrosslinking buffer (1% SDS, 0.1 M NaHCO 3 ) was added to the complexes overnight at 65 °C. DNA fragments were purified with a QIAquick Spin Kit (Qiagen, CA). For PCR, 2.5 μl from a 125-μl immunoprecipitated chromatin extraction and 250-μl input extraction, and 40 cycles of amplification were used. To assess differential FOXA1 binding at the heterozygous alleles, the MAMA (Mismatch Amplification Mutation Assays) PCR-based technique was used [26] . Reverse MAMA primers specific to each allele were designed with one mismatched nucleotide at the 3′ end [26] . The primers are listed in Supplementary Table 4 . Gene expression analysis MCF7 and BT474 total RNA was extracted using Trizol (Life Technologies) from untreated, oestrogen (10 nM)- or vehicle (DMSO)-treated cells. Residual DNA contaminants were removed by DNAse treatment (Ambion) and complementary DNA was synthesized using random primers as per manufacturers’ instructions (Life Technologies). All qPCRs were performed on a RotorGene 6000 (Corbett Research) with TaqMan Gene Expression assays (Hs00181213_m1 for IGFBP5 and Hs00907239_m1 for TFF1 ) and TaqMan Universal PCR master mix. All reactions were normalized against B-glucuronidase (MIM 611499; Catalogue No. 4326320E). For in vivo allele-specific gene expression, a primer outside of the rs4442975 SNP and its closest EcoRI restriction enzyme site and a primer outside of the SNP pos271557291 and its closest EcoRI site were first used to PCR amplify the EcoRI 3C product from BT474 cells. PCR-amplified products were cloned into pBLUNT empty vector (Life Technologies), then sequenced using the Sanger sequencing, which revealed the linkage between the two alleles ( Supplementary Fig. 10 ). BT474 genomic DNA was extracted using Qiagen DNeasy blood and tissue kit. BT474 total nuclear RNA was extracted using Trizol and cDNA synthesized using a gene-specific primer. PCR-amplified sequences from BT474 genomic DNA or cDNA were gel purified (Qiagen) and Sanger sequenced to measure the DNA and RNA levels of each allele. All experiments were conducted in biological triplicates and qPCR reactions as technical duplicates. The primers are listed in Supplementary Table 4 . eQTL analysis eQTL analyses were conducted in two studies: 123 normal breast tissue and 254 breast tumours from women in the Norwegian Breast Cancer Study (NBCS); all women were of Caucasian origin. The 123 normal breast tissue is a cohort of expression data from normal breasts biopsy ( n =74), reduction plastic surgery ( n =37) and adjacent normal ( n =12) (adjacent to tumour). Correlations between the two most likely causative SNPs (rs4442975 and rs6721996) and expression levels of nearby genes (500 kb upstream and downstream of the SNPs) were assessed using a linear regression model in which an additive effect on expression level was assumed for each copy of the rare allele. Calculations were carried out using the eMap library in R ( www.bios.unc.edu/~weisun/software/eMap ). The second eQTL analysis was based on 135 adjacent normal breast samples from women of Caucasian origin in the METABRIC study [27] . Matched gene expression (Illumina HT-12 v3 microarray) and germline SNP data that were either genotyped (Affymetrix SNP 6.0) or imputed (1000 Genomes Project, March 2012 data using IMPUTE version 2.0) were used. Statistical methods were identical to the NBCS analysis. How to cite this article: Ghoussaini, M. et al. Evidence that breast cancer risk at the 2q35 locus is mediated through IGFBP5 regulation. Nat. Commun. 5:4999 doi: 10.1038/ncomms5999 (2014).